All-linear time reversal by a dynamic artificial crystal The time reversal of pulsed signals or propagating wave packets has long been recognized to have profound scientific and technological significance. Until now, all experimentally verified time-reversal mechanisms have been reliant upon nonlinear phenomena such as four-wave mixing. In this paper, we report the experimental realization of all-linear time reversal. The time-reversal mechanism we propose is based on the dynamic control of an artificial crystal structure, and is demonstrated in a spin-wave system using a dynamic magnonic crystal. The crystal is switched from an homogeneous state to one in which its properties vary with spatial period a , while a propagating wave packet is inside. As a result, a linear coupling between wave components with wave vectors k ≈π/ a and k ′= k −2ππ/ a ≈ − π /a is produced, which leads to spectral inversion, and thus to the formation of a time-reversed wave packet. The reversal mechanism is entirely general and so applicable to artificial crystal systems of any physical nature. Mathematically, conversion between a time-dependent process f ( t ) and a time-reversed version of this process f (− t ) is a matter of trivial substitution; but the physical realization of such a transformation has profound significance. Not only are time-reversal mechanisms immensely powerful technological tools but their existence challenges our understanding of such fundamental notions as thermodynamic irreversibility, causality, and the perceived 'arrow' of time [1] . Artificial crystals are wave transmission systems which belong to a category of man-made media known as 'metamaterials'. A metamaterial is a synthetic material that has properties derived from an engineered mesoscopic (rather than atomic scale, or molecular) structuring. The defining feature of an artificial crystal is an 'artificial lattice' formed by wavelength-scale modulations in one or more of its material properties. Prominent examples include photonic [2] , [3] , [4] , [5] , [6] , [7] , [8] , [9] , [10] , [11] , [12] , [13] and magnonic [14] , [15] , [16] , [17] , [18] , [19] , [20] crystals; the former are optical systems and the latter operate in conjunction with spin waves (the propagating or standing magnetic oscillations—the quanta of which are known as magnons—which can be observed in ordered magnetic materials such as ferromagnets). The transmission spectra of artificial crystals abound with interesting features, most notably bandgaps: frequency intervals over which wave propagation is prohibited. The physical origin of these bandgaps lies in resonant wave-lattice interactions analogous to the atomic-scale Bragg scattering processes encountered in the context of X-ray or electron crystallography of natural crystals [21] . Research in the field of artificial crystals began with the development of static systems; crystals having a permanent artificial lattice defined at the time of fabrication. Recently, however, a new class of dynamic artificial crystals has emerged. A dynamic artificial crystal has a lattice with properties which can be modified while a wave packet propagates inside it [7] , [8] , [9] , [10] , [11] , [12] , [13] , [14] , [15] . It has been suggested that such systems—which offer unique opportunities for the manipulation of propagating waves—may provide linear means to perform spectral transformations, including time reversal [2] , [3] , [12] , [22] , [23] , which, until now, have only been possible through nonlinear mechanisms [22] , [23] , [24] , [25] . Several linear methods of time reversal in dynamic photonic crystals based on, for example, Bloch oscillations [10] and refractive index- or loss-tuning of coupled cavity waveguides [2] , [3] have been proposed theoretically, but none has been observed experimentally. The results we report in this paper constitute both the first demonstration of the spectral transformation of a waveform of finite spectral width using a dynamic artificial crystal, and the first experimental realization of all-linear time reversal of a propagating wave packet. The time-reversal mechanism we propose—which is a principle of universal application to waves of any nature—is predicated on the manipulation of a dynamic artificial crystal structure on a timescale comparable with the temporal characteristics of a wave packet travelling through it. Its underlying physical basis is a linear non-stationary process, making it entirely distinct from known nonlinear mechanisms of time reversal (for example, optical four-wave mixing [22] , [23] , [24] ). We demonstrate our proposed time-reversal mechanism experimentally using spin waves in a dynamic magnonic crystal (DMC) [14] ( Fig. 1a ). The use of spin-wave systems as model environments for the study of general wave and quasi-particle phenomena is well established [25] , [26] , [27] , [28] , [29] , [30] , [31] and, indeed, in this context, magnonic crystals are increasingly recognized as an important route to fundamental understanding of wave dynamics in metamaterials [14] , [15] , [16] , [17] , [18] , [19] , [20] . The process of time reversing a signal is equivalent, in the frequency domain, to an inversion of its spectrum about a certain reference frequency [2] . Accordingly, for clarity, we reveal our time-reversal mechanism through two separate experiments. The first demonstrates frequency inversion of quasi-monochromatic signals and the second demonstrates time reversal of complex waveforms. 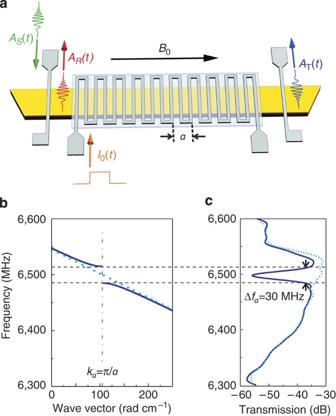Figure 1: Experimental dynamic magnonic crystal (DMC) system. (a) The DMC comprises a planar current-carrying meander structure with 20 periods of lattice constanta=300 μm (10 shown), positioned close to the surface of an Yttrium Iron Garnet thin-film spin-wave waveguide (thickness 5 μm, width 2 mm). Two spin-wave antennae are arranged on the surface of the film 8 mm apart: one to launch a spin-wave signal, amplitudeAS(t) and to detect the signalAR(t) reflected by the DMC, and a second to detect the signalAT(t) transmitted through it. (b) Theoretical spin-wave dispersion relationship for the waveguide with no applied current (dotted, light blue) and with a static current of 1 A in the meander structure (solid curve, dark blue). (c) Experimental spin-wave transmission characteristics with no current (dotted, light blue) and with a current of 1 A (solid curve, dark blue) applied to the meander structure. Application of the current leads to the formation of a bandgap of width approximately Δfa=30 MHz, centred onfa=6,500 MHz. Figure 1: Experimental dynamic magnonic crystal (DMC) system. ( a ) The DMC comprises a planar current-carrying meander structure with 20 periods of lattice constant a =300 μm (10 shown), positioned close to the surface of an Yttrium Iron Garnet thin-film spin-wave waveguide (thickness 5 μm, width 2 mm). Two spin-wave antennae are arranged on the surface of the film 8 mm apart: one to launch a spin-wave signal, amplitude A S ( t ) and to detect the signal A R ( t ) reflected by the DMC, and a second to detect the signal A T ( t ) transmitted through it. ( b ) Theoretical spin-wave dispersion relationship for the waveguide with no applied current (dotted, light blue) and with a static current of 1 A in the meander structure (solid curve, dark blue). ( c ) Experimental spin-wave transmission characteristics with no current (dotted, light blue) and with a current of 1 A (solid curve, dark blue) applied to the meander structure. Application of the current leads to the formation of a bandgap of width approximately Δ f a =30 MHz, centred on f a =6,500 MHz. Full size image Experimental DMC system A thin-film Yttrium Iron Garnet (YIG) spin-wave waveguide forms the basis for our one-dimensional DMC system. The waveguide is biased by a static magnetic field B 0 parallel to the direction of spin-wave propagation (see Methods section for further details and justification). Adjacent to the surface of the YIG is a planar metallic meander structure [14] , [32] with 20 periods of lattice constant a =300 μm ( Fig. 1a ). If a current is applied to the meander structure, the Oersted field that results (amplitude Δ B ) spatially modulates the waveguide's magnetic bias field and leads to the formation of a magnonic bandgap in its transmission characteristics. Microstrip antennae are positioned at each end of the system: an input antenna to launch a spin-wave signal A S ( t ) and to detect the signal A R ( t ) reflected by the DMC, and an output antenna to receive the signal A T ( t ) transmitted through it. Figure 1b,c provides a quantitative illustration of the difference between the characteristics of the system with and without a current flowing in the DMC meander structure. In the absence of an applied current, the meander structure has negligible influence on spin-wave transmission through the waveguide (dotted line, Fig. 1c ) and the dispersion relationship f ( k ) (dotted line, Fig. 1b ) is continuous. Under these conditions, the DMC is said to be 'off'. Note that the negative slope of the dispersion curve is a practical detail that has no bearing on the results we go on to describe (see Methods section for elucidation). The application of a static current of 1 A to the meander structure results in the formation of a magnonic bandgap of width approximately Δ f a =30 MHz, centred on the DMC's Bragg resonance frequency f a =6,500 MHz, which corresponds to the Bragg wave vector k a =π/ a =105 rad cm −1 . This bandgap manifests itself as a deep rejection band in the experimental spin-wave transmission characteristics (solid line, Fig. 1c ) and appears as a discontinuity in the dispersion relationship ( Fig. 1b ). Frequency inversion experiments Frequency inversion was studied in the following manner. With the DMC 'off', a spin-wave signal packet of carrier frequency f S , duration 200 ns (bandwidth 5 MHz), and amplitude A S ( t ) was launched into the waveguide. After a delay, a rectangular current pulse I 0 ( t ) of duration 25 ns was supplied to the meander structure ( Fig. 1a ). Timing parameters were chosen so that the packet was contained within the DMC at the time of the application of the current pulse and its spectrum lay entirely within the bandgap. The carrier frequency f S of the packet was varied over a range of ±15 MHz about the resonance frequency f a =6,500 MHz while its power was maintained at <1 mW. The spectrum of the reflected wave packet A R ( t ) was captured using a spectrum analyser. The spatially modulated magnetic field created in the DMC by the current pulse I 0 ( t ) leads to a strong coupling between (initially independent) spin waves having wave vectors k and k ′= k ±2 k a . This coupling is especially efficient for k ≈ k a , k ′= k −2 k a ≈− k a when the frequencies of the coupled waves are close to each other, and lie within the bandgap of the DMC. By analogy with a system of two coupled oscillators [33] , the DMC-induced coupling leads to a transfer of energy between the initially excited signal wave of wave vector k S and a reflected wave of wave vector. After a certain time ( ∼ 25 ns under the conditions of our experiment), a substantial fraction of the energy is transferred from the signal ( k S ) to the reflected ( k R ) wave. If the current, and therefore the field modulation, is switched off at this time, removing the coupling, the two waves become once again independent and the reflected wave propagates back towards the input antenna. The reflected frequency f R = f ( k R ) can be determined using a linear Taylor expansion of the dispersion relationship f ( k ) about k S ≈ k a . The incident signal frequency is given by f S = f ( k S )≈ f a + v ( k S − k a )/(2π), where f a = f ( k a ) is the centre frequency of the DMC bandgap and v =2πd f ( k a )/d k a is the spin-wave group velocity. Using equation (1) and the inversion symmetry of the dispersion curve, the frequency of the reflected wave can be written as f R ≈ f a − v ( k S − k a )/(2π). Thus, the frequencies of the counter-propagating incident and reflected waves are connected by the simple relation that is, they are inverted with respect to the centre of the bandgap f a . 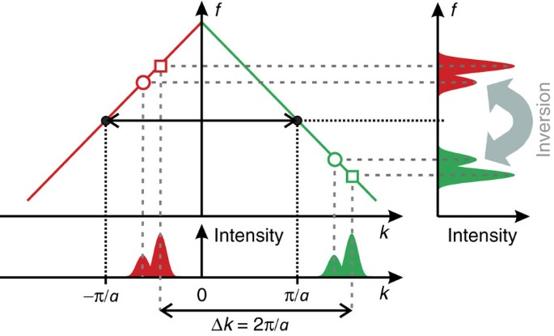Figure 2: Schematic diagram illustrating frequency inversion by the dynamic magnonic crystal. The diagonal lines (green and red) represent the spin-wave dispersion curve. Incident signal waves have positive wave vectors (green section) and those reflected by the DMC have negative wave vectors (red section). These two groups of waves are counter propagating. Black dots mark the reference frequencyfalying in the centre of the bandgap and corresponding to the Bragg wave vectors ±ka=±π/a. The green open circle and square illustrate two spectral components of an incident signal waveform. The spatially periodic magnetic modulation of the waveguide's magnetic bias field brought about by the application of the current pulse to the DMC meander structure couples these components to corresponding components of a reflected waveform (red open circle and square). The difference between the wave vectors of the signal and reflected waves is fixed by the lattice constantaof the DMC so that thek-spectrum of the reflected waveform is uniformly shifted to the left by Δk=2π/a=2ka(lower panel). This uniform shift ink-space results in spectral inversion in the frequency domain (right panel). The reference frequencyfa(black dots) is not shifted and provides the axis of inversion. This process of dynamic reflection and linear frequency inversion is illustrated schematically in Figure 2 . Figure 2: Schematic diagram illustrating frequency inversion by the dynamic magnonic crystal. The diagonal lines (green and red) represent the spin-wave dispersion curve. Incident signal waves have positive wave vectors (green section) and those reflected by the DMC have negative wave vectors (red section). These two groups of waves are counter propagating. Black dots mark the reference frequency f a lying in the centre of the bandgap and corresponding to the Bragg wave vectors ± k a =±π/ a . The green open circle and square illustrate two spectral components of an incident signal waveform. The spatially periodic magnetic modulation of the waveguide's magnetic bias field brought about by the application of the current pulse to the DMC meander structure couples these components to corresponding components of a reflected waveform (red open circle and square). The difference between the wave vectors of the signal and reflected waves is fixed by the lattice constant a of the DMC so that the k -spectrum of the reflected waveform is uniformly shifted to the left by Δ k =2π/ a =2 k a (lower panel). This uniform shift in k -space results in spectral inversion in the frequency domain (right panel). The reference frequency f a (black dots) is not shifted and provides the axis of inversion. 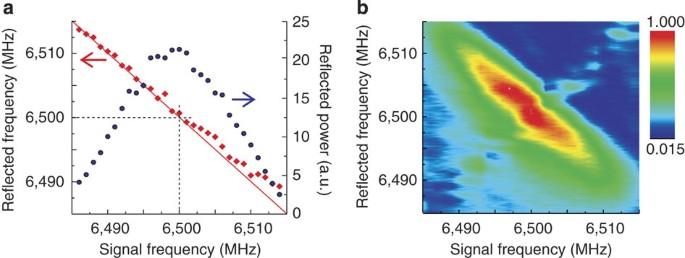Figure 3: Experimental demonstration of frequency inversion by the dynamic magnonic crystal. (a) When the carrier frequency of the incident spin-wave signal packet is detuned from the resonance value of 6,500 MHz (the bandgap centre frequency), the frequency of the reflected signal is inverted about this value (left ordinate axis, red diamonds). The solid red line is the theoretical curve of equation (2). The efficiency of the reflection process (right ordinate axis, blue circles) is maximum at the resonance condition and decreases symmetrically with detuning. (b) Two-dimensional map of reflected signal spectra as a function of the incident signal carrier frequencyfS(31 spectra taken at 1 MHz intervals offS). Dark red is indicative of the highest signal intensities, dark blue the lowest; the intervening colour scale is linear. Frequency inversion is clearly demonstrated by the diagonal stripe of high signal intensity with a negative slope (running from the upper left to the lower right corner of the figure). The weak diagonal stripe with a positive slope (from the lower left to the upper right corner) is due to weak conventional (that is, frequency conserving) reflection from inhomogeneities in the spin-wave waveguide. Full size image Experimental demonstration of frequency inversion in the DMC system is shown in Figure 3 . The efficiency of the process is maximal in the case of f S = f a , and decreases symmetrically with positive and negative detuning ( Fig. 3a ). Figure 3b shows the spectrum of the reflected signal as a function of the incident signal carrier frequency f S . The spectral width of the reflected packet is of order 5 MHz—the bandwidth of the 200 ns input pulse—indicating that no significant spectral broadening is introduced in the dynamic reflection process. Figure 3: Experimental demonstration of frequency inversion by the dynamic magnonic crystal. ( a ) When the carrier frequency of the incident spin-wave signal packet is detuned from the resonance value of 6,500 MHz (the bandgap centre frequency), the frequency of the reflected signal is inverted about this value (left ordinate axis, red diamonds). The solid red line is the theoretical curve of equation (2). The efficiency of the reflection process (right ordinate axis, blue circles) is maximum at the resonance condition and decreases symmetrically with detuning. ( b ) Two-dimensional map of reflected signal spectra as a function of the incident signal carrier frequency f S (31 spectra taken at 1 MHz intervals of f S ). Dark red is indicative of the highest signal intensities, dark blue the lowest; the intervening colour scale is linear. Frequency inversion is clearly demonstrated by the diagonal stripe of high signal intensity with a negative slope (running from the upper left to the lower right corner of the figure). The weak diagonal stripe with a positive slope (from the lower left to the upper right corner) is due to weak conventional (that is, frequency conserving) reflection from inhomogeneities in the spin-wave waveguide. Full size image Time-reversal experiments The frequency inversion described by equation (2) directly implies reversal of the time profile of the signal packet [2] . This can be seen by writing the time profile of the incident waveform as a Fourier series A S ( t ) ∼ ∑ Δ f exp( i 2πΔ ft ), where Δ f = f − f a is the frequency detuning of a given spectral component from the bandgap centre frequency f a . In the process of frequency inversion, the sign of the detuning Δ f inverts, and thus the dynamically reflected signal has a reversed time profile A R ( t ) ∼ ∑ Δ f exp(− i 2πΔ f t ) ∼ A S (− t ). To observe the effect of time reversal experimentally, a train of two input spin-wave pulses with carrier frequency f S = f a =6,500 MHz, 70 ns duration, and spacing 40 ns was used. 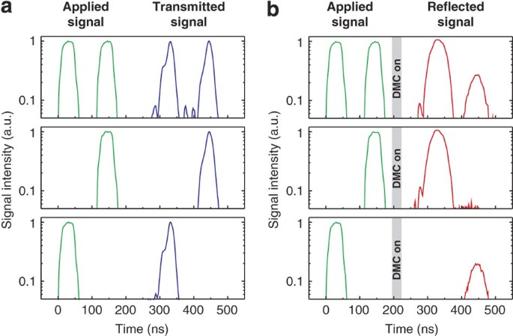Figure 4: Experimental demonstration of time reversal by the dynamic magnonic crystal. A train of two spin-wave pulses (70 ns wide and spacing 40 ns) with carrier frequencyfS=6,500 MHz was applied to the input antenna. The applied signals shown (green) are the envelopes of those supplied by the microwave generator. (a) The transmitted spin-wave signals with no current applied to the DMC meander structure appear after a delay of∼300 ns (upper frame, blue). When the first of the two input pulses is switched off, the first transmitted pulse is absent (middle frame) and the same is true for the second pulse (lower frame). (b) The reflected spin-wave signals obtained after a brief interval of magnetic field modulation within the DMC (shaded area shows the time interval of the current pulse applied to the meander structure). In the case that two spin-wave pulses are applied, two corresponding reflected pulses are observed (upper frame, red). When the first of the two pulses is switched off, the second reflected pulse is absent (middle frame), and vice versa (lower frame), confirming time reversal. Figure 4a shows—for reference—time profiles of input (green) and transmitted (blue) signals detected in the absence of DMC activation. Here, if the first spin-wave pulse is switched off (middle frame), the first pulse in the transmitted signal disappears. Similarly, the switching off of the second pulse (lower frame) leads to the disappearance of the second transmitted envelope. Figure 4: Experimental demonstration of time reversal by the dynamic magnonic crystal. A train of two spin-wave pulses (70 ns wide and spacing 40 ns) with carrier frequency f S =6,500 MHz was applied to the input antenna. The applied signals shown (green) are the envelopes of those supplied by the microwave generator. ( a ) The transmitted spin-wave signals with no current applied to the DMC meander structure appear after a delay of ∼ 300 ns (upper frame, blue). When the first of the two input pulses is switched off, the first transmitted pulse is absent (middle frame) and the same is true for the second pulse (lower frame). ( b ) The reflected spin-wave signals obtained after a brief interval of magnetic field modulation within the DMC (shaded area shows the time interval of the current pulse applied to the meander structure). In the case that two spin-wave pulses are applied, two corresponding reflected pulses are observed (upper frame, red). When the first of the two pulses is switched off, the second reflected pulse is absent (middle frame), and vice versa (lower frame), confirming time reversal. Full size image The signal reflected by the DMC is shown in Figure 4b (red). When both spin-wave pulses are applied, two corresponding reflected pulses are observed (upper frame). Here, however, unlike in the case of the transmitted signal, the switching off of the first pulse results in the disappearance of the second reflected signal (middle frame). The corresponding situation when the second pulse is absent—the disappearance of the first reflected signal—is indicated in the lower frame. This behaviour provides direct evidence of time reversal. The relative intensity of the two reflected signals in the upper frame of Figure 4b is consistent with the fact that, in the process of dynamic reflection, the second reflected pulse has a longer propagation time and thus—due to dissipation—is attenuated more significantly than the first one. In this paper, we have demonstrated that the fast manipulation of an artificial crystal structure while a propagating wave packet is inside it leads to a previously unforeseen linear coupling between the wave packet's spectral components. The coupling occurs between spectral components that correspond to counter-propagating waves with wave vectors related by the lattice constant a of the crystal: k ≈π/ a and k ′= k −2π/ a ≈−π /a and accordingly, gives rise to an inversion of the incident packet's spectrum about the centre frequency of the crystal's bandgap, and the formation of a time-reversed wave packet. The work reported here establishes that dynamic phenomena in artificial crystals can provide a substitute for the nonlinear mechanisms traditionally used to perform complex spectral transformations such as time reversal. As the overwhelming majority of real materials exhibit only weak nonlinearity, we suggest that this capability may provide an enabling route towards the development of low-power signal and information processing systems with complex functionalities. Established time-reversal mechanisms that operate by phase-matched nonlinear mixing typically have a bandwidth which is restricted by that of a resonant enhancement or absorption phenomenon in the signal transmission medium. The linear time-reversal mechanism proposed here operates by virtue of a dynamic geometrical interaction between an incident wave packet and an artificial crystal lattice and, accordingly, is subject to no such bandwidth constraint. Although we stress that the key result presented in this article is an entirely general one, it is nevertheless the case that our experimental results also have significance as a specific and exciting development in the field of magnonics. Magnonics [26] , [31] , the study of spin-wave propagation phenomena in magnetic films and nanostructures, is increasingly widely recognized as an important route to technological opportunity in the field of spintronics [30] . Spintronics [34] , [35] , [36] , [37] , or spin transport electronics, is concerned with the development of functional electronic devices which exploit not just the charge-carrying properties of the electron but also its intrinsic magnetic moment or 'spin'. One of the foremost aspirations of contemporary spintronics is the development of an integrated spin-information platform combining signal processing, transport, and storage. In this context, magnonics has a great deal of potential; not only are spin waves capable of transporting spin angular momentum but their small group velocities, short wavelengths, and highly tunable dynamic properties make them well suited to the requirements of nanoscale device development [25] , [26] , [27] , [28] , [29] , [30] , [31] . The results presented in this article demonstrate that magnonic crystals are capable of providing previously unanticipated spin-information processing functionality. DMC system An Yttrium Iron Garnet (YIG) thin-film spin-wave waveguide was chosen as the basis for our one-dimensional DMC system. Monocrystalline YIG has the narrowest magnetic resonance linewidth of any known material (typically ∼ 0.04 mT in thin-film samples), allowing spin-wave propagation over centimetre distances and making it the ideal choice for experimental spin-wave studies. Our waveguide is a strip of YIG film (of width 2 mm, thickness 5 μm, and saturation magnetization approximately μ 0 M 0 =0.175 mT), which was grown by high-temperature liquid-phase epitaxy on a Gallium Gadolinium Garnet substrate (YIG surface normal parallel to the <111> crystallographic axis). The DMC comprises a planar metallic meander structure [14] , [32] with 20 periods of lattice constant a =300 μm, separated from the surface of the waveguide by a 100 μm glass spacer layer ( Fig. 1a ). This spacer layer is used to prevent direct inductive interaction between the metallic structure and propagating spin waves in the YIG. The width of the metallic structure and the glass spacer layer is large compared with the width of the waveguide [14] . A current pulse I 0 ( t ) of amplitude ∼ 1 A applied to the meander structure creates a periodic Oersted field of amplitude Δ B ∼ 1 mT which spatially modulates the waveguide's static magnetic bias field B 0 =180 mT. Two microstrip antennae are positioned 8 mm apart, ∼ 1 mm from each end of the DMC: an input antenna to launch a spin-wave signal A S ( t ) and to detect the signal A R ( t ) reflected by the DMC, and an output antenna to receive the signal A T ( t ) transmitted through it. Several dynamically distinct types of spin waves can propagate in YIG films. These types are categorized according to the angle between their propagation direction and the magnetic bias field. The in-plane, on-axis orientation of the static bias field used in the experiment ( Fig. 1a ) corresponds to the propagation of backward volume magnetostatic spin waves (BVMSW) [26] , [31] . BVMSW feature a dispersion curve f ( k ) with a negative slope as indicated in Figure 1b, but it is stressed that this practical detail has no bearing on the entirely general result we describe. BVMSW were used in the experimental investigations as they are reciprocal waves and are readily excited and received by inductive microstrip antennae [26] . Frequency inversion experiments Frequency inversion experiments involved launching a spin-wave signal packet of carrier frequency f S , duration 200 ns (bandwidth 5 MHz) and amplitude A S ( t ) into the waveguide with the DMC 'off'. The 200 ns packets were produced using an (externally triggered) Agilent 8673B Synthesized Signal Generator (frequency range 2–26.5 GHz) and applied by means of a broadband 3 port (input, output, and return) microwave Y-circulator. After a delay, a rectangular current pulse I 0 ( t ) of duration 25 ns, amplitude ∼ 1 A, and rise/fall time <5 ns was supplied to the DMC meander structure from an Agilent 8114A High Power Pulse Generator ( Fig. 1a ) through a matching network. To generate the data of Figure 3, the carrier frequency f S of the input packet was varied over a range of ±15 MHz about the bandgap centre frequency f a =6,500 MHz of the DMC. Timing parameters (all controlled by a single programmable pulse generator) were such that, in all experiments, the packet was contained within the magnonic crystal at the time of the application of the current pulse to the meander structure, and its spectrum lay entirely within the DMC bandgap. Throughout, the input microwave signal power was maintained below 1 mW (two orders of magnitude lower than that known to be required to observe the effects of nonlinear terms in YIG's microwave susceptibility [26] ). The spectrum of the reflected wave packet A R ( t ) was captured by means of the return signal port of the Y-circulator using a spectrum analyser (Agilent E4446A, 3 Hz–44 GHz). The experiments were conducted with a 500 μs repetition rate. Time-reversal experiments In our time-reversal experiments, the spin-wave input signal was a train of two pulses with carrier frequency f S = f a =6,500 MHz, 70 ns duration, and spacing 40 ns. As in the frequency inversion investigation, the 1 mW signal pulses were produced using an externally triggered Agilent 8673B Generator and applied using a broadband 3 port microwave Y-circulator with the DMC 'off'. A current pulse identical in amplitude and duration to that used in the frequency inversion experiments was used to time reverse the signals. To capture the data of Figure 4 , the Y-circulator return port at the spin-wave input antenna (connected to the spectrum analyser in the frequency inversion experiments) was provided to a digital storage oscilloscope (Agilent InfiniVision DSO7034A, 350 MHz) through an amplifier and broadband detector diode. A second channel of the oscilloscope was connected to the output antenna through a similar amplification and rectifying circuit. Again, the experiments were conducted with a 500 μs repetition rate. How to cite this article: Chumak, A. V. et al . All-linear time reversal by a dynamic artificial crystal. Nat. Commun. 1:141 doi: 10.1038/ncomms1142 (2010).